Interferon-induced transmembrane protein-3 genetic variant rs12252-C is associated with severe influenza in Chinese individuals The SNP rs12252-C allele alters the function of interferon-induced transmembrane protein-3 increasing the disease severity of influenza virus infection in Caucasians, but the allele is rare. However, rs12252-C is much more common in Han Chinese. Here we report that the CC genotype is found in 69% of Chinese patients with severe pandemic influenza A H1N1/09 virus infection compared with 25% in those with mild infection. Specifically, the CC genotype was estimated to confer a sixfold greater risk for severe infection than the CT and TT genotypes. More importantly, because the risk genotype occurs with such a high frequency, its effect translates to a large population-attributable risk of 54.3% for severe infection in the Chinese population studied compared with 5.4% in Northern Europeans. Interferon-induced transmembrane protein-3 genetic variants could, therefore, have a strong effect of the epidemiology of influenza in China and in people of Chinese descent. There is strong evidence that the interferon-induced transmembrane protein-3 (IFITM3) protein is a virus restriction factor mediating cellular resistance to influenza viruses and other viruses that enter cells via the acidic endosome [1] , [2] , [3] . The importance of IFITM3 in influenza virus infection was determined by Everitt et al. [4] who showed that severity of influenza virus infection was greatly increased in IFITM3 knockout mice compared with wild-type animals. In humans, the rare SNP rs12252-C allele of IFITM3 truncates the protein, leading to reduced restriction of virus replication in vitro [4] , [5] . In Northern European patients infected and hospitalized with seasonal influenza or pandemic influenza A (H1N1)pdm/09 (pH1N1/09) virus, there was an increased homozygosity of the minor C allele of SNP rs12252 in IFITM3 (5.7 versus 0.3%, n =53). This was the first direct evidence for a host genetic influence on influenza severity in humans. However, because of the rarity of the susceptibility allele (minor allele frequency=0.034) in people of Northern European descent, the overall effect on the severity of pandemic or seasonal influenza virus in the population is likely to be small. However, the frequency of the IFITM3 rs12252 susceptibility allele is known to be much higher in Han Chinese (minor allele frequency=0.5). Here we examine the influence of this polymorphism on severity of influenza A virus infection in Chinese patients. We found a striking high frequency of the CC genotype among patients in China infected by the 2009 pandemic H1N1 virus with severe illness compared with mild infection and the healthy Han Chinese. This implies that the presence of the variant IFITM3 gene influences disease severity rather than susceptibility to infection. Furthermore, using statistic analysis tools, we estimated that patients with the CC genotype have a sixfold greater risk of severe infection compared with those with the CT and TT genotype. The much higher level of CC allele at population level in Han Chinese compared with Caucasians may place the Chinese at a higher risk for developing severe illness upon influenza virus infection. Clinical and laboratory characteristics of study subjects During the 2009 pandemic, hospitals in China admitted patients with severe infection, but also, unusually, patients with mild infection, who under normal circumstances would not require hospitalization. This ‘open-door’ policy provided a unique opportunity to capture a relatively unselected group of patients with divergent outcomes, observed and managed under similar clinical conditions. In this cohort, 83 patients fulfilled the criteria for inclusion (influenza pdmH1N1/09 infection confirmed by viral genome PCR assay, able to give informed consent) and exclusion (use of corticosteroids or any other immunosuppressants for 1 month before or during sampling, coexisting illnesses, pregnancy, positive bacterial cultures from respiratory tract secretions/sputum or blood at any point during hospital admission). Blood was obtained 2 or 3 days after admission and the progress of patients was observed throughout the duration of their hospital stay. At the point of discharge, patients were divided into those with ‘mild’ and ‘severe’ disease by perusal of the clinical data over the entire course of their stay. Mild disease ( n =51) was defined as those who reported symptoms (fever, cough, headache and lethargy) only, and whose circulating leukocyte profile (total leukocyte, lymphocytes and neutrophils) was normal throughout the hospital stay. Patients with severe disease ( n =32) were those who reported the symptoms described above, but deteriorated and developed pneumonic consolidation and/or bilateral infiltrates on chest radiograph with or without respiratory failure (defined as PaO 2 /FiO 2 <200 mm Hg), or respiratory failure with disseminated intravascular coagulopathy or renal failure (only 1 of the 32 patients). All the patients (32/32) in severe group used Oseltamivir, and 38/51 of patients in mild group were given Oseltamivir. No patients developed pleural effusion or empyema. Six patients were mechanically ventilated and all of these were among the thirteen severely infected patients who died. 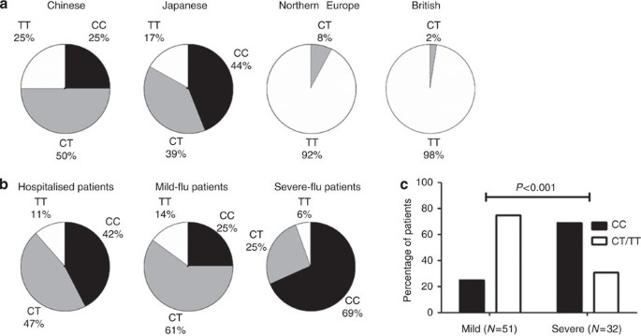Figure 1: C allele at SNP 12252 associated with disease severity in acutely influenza A (H1N1)pdm/09 infected Chinese individuals. (a) Allele frequencies were obtained from the 1,000 genomes project: allele frequencies vary significantly among different populations. (b) Allele frequencies obtained from Influenza A pH1N1/09 confirmed patients from Beijing You’an Hospital. (c) Proportion of mild versus severe flu patients carrying CC or CT/TT genotype with confirmed Influenza A pH1N1/09 infection from Beijing You’an Hospital. Demographic data are shown in Table 1 . Table 1 Clinical and laboratory characteristics. Full size table The C allele at SNP 12252 was associated with disease severity We sequenced 300 base pairs of the IFITM3 locus encompassing SNP rs12252 in these 83 pH1N1/09 infected individuals. 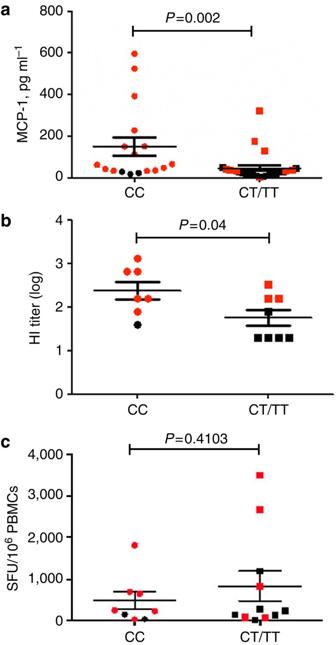Figure 2: C allele at SNP 12252 is associated with higher serum MCP-1 and antibody level, the data points were color coded in the figure for severe (red) and mild (black) disease. (a) Serum MCP-1 levels in patients with CC and CT/TT genotype. (b) Influenza A virus (H1N1)pdm/09-specific antibody levels in patients with CC genotype and CT/TT genotype. (c). Overall influenza A virus (H1N1)pdm/09-specific T-cell responses in patients with CC genotype and CT/TT genotype. Of these, 42.17% carried the CC genotype, a higher frequency than in the Han Chinese in the 1,000 genomes sequence database (25.38% CC genotype; ( P =0.0001, χ 2 -test)) ( Table 2 , Fig. 1a and b ). We then stratified hospitalized patients into mild and severe, based on clinical assessment ( Table 1 ). Mildly ill individuals did not have significantly different allele frequencies compared with the Han Chinese population ( P =0.36, χ 2 -test). Severely ill patients had a significantly different allele frequency compared with the mild cases ( P =0.000007, χ 2 -test) and compared the general Han Chinese population ( P =0.000005, χ 2 -test). A significantly higher frequency of the homozygous CC genotype was found in patients who developed severe illness (68.75%, P =0.0001) ( Table 2 , Fig. 1b and c ). Ten of the thirteen patients who died carried the CC genotype. Table 2 Allele and genotype frequencies of IFITM3 rs12252 in Chinese pH1N1-infected patients and the population. Full size table Figure 1: C allele at SNP 12252 associated with disease severity in acutely influenza A (H1N1)pdm/09 infected Chinese individuals. ( a ) Allele frequencies were obtained from the 1,000 genomes project: allele frequencies vary significantly among different populations. ( b ) Allele frequencies obtained from Influenza A pH1N1/09 confirmed patients from Beijing You’an Hospital. ( c ) Proportion of mild versus severe flu patients carrying CC or CT/TT genotype with confirmed Influenza A pH1N1/09 infection from Beijing You’an Hospital. Full size image The recessive model has the largest odds ratio We analysed the association of rs12252 with severe infection by comparing against the mildly infected individuals assuming different genetic models ( Table 3 ). We could explicitly assess whether one (dominant) or two copies (recessive) of the C allele increase risk of severe infection, as well as whether the risk increase is significant assuming multiplicative ( r -fold increase for CT, r 2 for CC genotype) or additive models ( r -fold increase for CT, 2 r -fold for CC genotype). All models apart from the dominant model show significant association to severe infection with the recessive model having the largest odds ratio. In particular, under the multiplicative model, the carriers of the C allele showed a threefold increase in risk for severe infection compared with carriers of the T allele (multiplicative model P -value=7.936 × 10 −4 , odds ratio=3.42, 95% confidence interval 1.63–7.17). Under the recessive model, homozygotes for the C allele were estimated to have a larger, sixfold greater risk for severe infection compared with heterozygotes and homozygotes for the T allele (recessive model P -value=2.01 × 10 −4 , odds ratio=6.43, 95% confidence interval 2.42–17.1). Table 3 Association of rs12252 to severe infection under different genetic models. Full size table Elevated serum levels of monocyte chemotactic protein-1 in patients with CC genotype Together these analyses suggest that the CC variant does not increase the chance of initial virus infection but is associated with severity of the illness, although a larger study including another population is required to prove this definitively. The cytokine monocyte chemotactic protein-1 (MCP-1) is elevated in several viral infections and levels were raised in the lungs of IFTIM3 knockout mice after influenza virus infection [4] . When we grouped the patients by IFTIM3 genotype, we found significantly elevated serum levels of MCP-1 in the patients with the CC genotype compared with patients with CT or TT genotype ( P =0.002) ( Fig. 2a ). We also found a higher level of influenza A pH1N1/09-specific antibodies in patients with the CC genotype ( P =0.04) ( Fig. 2b ). These data indicate that the CC genotype is associated with a more overt immune response possibly due to higher viral (antigen) load. We did not observe any significant differences in T-cell responses, measured by interferon-gamma ELISpot assays with peptides spanning the whole virus proteome, between patients with and without the CC genotype ( Fig. 2c ). Figure 2: C allele at SNP 12252 is associated with higher serum MCP-1 and antibody level, the data points were color coded in the figure for severe (red) and mild (black) disease. ( a ) Serum MCP-1 levels in patients with CC and CT/TT genotype. ( b ) Influenza A virus (H1N1)pdm/09-specific antibody levels in patients with CC genotype and CT/TT genotype. ( c ). Overall influenza A virus (H1N1)pdm/09-specific T-cell responses in patients with CC genotype and CT/TT genotype. Full size image Our data show that the IFITM3 -SNP, rs12252 is associated with disease severity following influenza virus infection in the Chinese population. IFITM3 restricts the replication of influenza virus infection in humans and mice; however, IFITM3 CC homozygotes are more likely to suffer severe respiratory pathology in both UK Caucasians and Han Chinese. Larger scale studies are urgently required to determine whether genotyping for IFITM3-sn12252 in Han Chinese and other Asian patients infected with influenza virus can predict those who might progress to severe disease early in their infection. In these it might be possible to improve their prognosis by early intensification of their treatment. In addition, genotyping should be considered when selecting patients for clinical trials and for studies of influenza virus infection, especially those involving virus challenges with a low pathogenic virus. SNP typing in China costs ~US$8 per sample, and this could be done in most large hospital laboratories. The IFITM3 effect is not dependent on influenza virus subtype, restricting both influenza A and B viruses [4] . In this study, we showed an effect on severity of a low pathogenic influenza A virus in humans. For a more pathogenic virus such as the avian H5N1 influenza virus that has a high fatality rate (59%) [6] , it is possible that the CC genotype could enhance the disease or that the virulent virus overrides the usual protective effects of the CT and TT genotypes. This will need further study. Future studies will also ask whether the disease course differs between severely infected patients who have the CC genotype and those with the CT or TT genotypes. It is intriguing that the CC genotype [4] is rare in Northern Europeans and common in Asian populations. As many other viral infections are restricted by IFITM3 in vitro , including severe acute respiratory syndrome (SARS) coronavirus, Dengue virus and West Nile virus [1] , [7] the high population allele frequencies may have been influenced by complex virus exposures. An estimate of how many individuals would develop severe infection specifically due to their CC genotype is given by the population-attributable risk (PAR). This largely depends on the frequency of the risk genotype in the population. As the risk genotype occurs at high frequency in the Chinese population, its effect translates into a large PAR, accounting for 54.25% of severe infection. This is much larger than the corresponding PAR of 5.39% in Northern Europeans, and implies that the incidence of severe influenza infection might be higher in Chinese than in Northern Europeans. This should be explored in future epidemiological studies. In conclusion, our data clearly extend the earlier observation in a European cohort that the IFTM3-rs12252CC genotype is significantly associated with influenza severity. The association is primarily with severity of disease rather than susceptibility to infection, although larger studies are required to prove this specific association. IFITM3 may have an important role in virus replication and dissemination following the initial infection. The much higher level of the CC genotype in the Han Chinese population compared with Caucasians may place the Chinese at a higher risk for developing severe illness upon influenza infection. It is not known whether those who are more severely infected with influenza virus are more likely to spread the infection. If this is the case, the high frequency of the C allele in Asian populations may influence the epidemiology of influenza. Subjects Patients were recruited from Beijing You’an Hospital, Beijing, between June 2009 and January 2010. The study was approved by the Institutional Review Board of Beijing You’An Hospital. Written informed consent was obtained from all patients. Sequencing and genotyping of rs12252 Genomic DNA was extracted from peripheral blood mononuclear cell using the PureGene DNA Isolation kit (Gentra Systems, Minneapolis, MN, USA). The region encompassing the human IFITM3 rs12252 sequences were amplified by polymerase chain reaction. The amplification was performed using the following forward and reverse primers: 5′-GGAAACTGTTGAGAAACCGAA-3′ and 5′- CATACGCACCTTCACGGAGT-3′ (Beijing Institute of Genomics(BGI),Shenzhen, China). The PCR products were purified and sequenced on an Applied Biosystems 3730xl DNA Analyser (GATC Biotech). Single-nucleotide polymorphisms were identified using Chromas (Technelysium Pty Ltd) at the BGI, Shenzhen, China. MCP-1 quantification EDTA-separated serum was stored at −80 °C until analysis. MCP-1 was analysed using a Human Cytokine multiplex assay (Bio-Rad, USA) and Luminex multi-analytic profiling technology (Bio-Rad, USA) according to the manufacturer’s instructions as described previously [8] . In brief, serum samples were diluted 1 in 4 with sample diluent, while standards were reconstituted in standard diluent. Standards and samples were incubated with the magnetic beads in a 96-well plate for 30 min at room temperature. After this, detection antibody was added to each well, and incubated at room temperature for a further 30 min. Streptavidin-PE was used as the fluorochrome for antibody detection. Using Bio-Plex Manager software version 6.0, standard Luminex maintenance procedures were performed, and Bio-Plex CAL1 and CAL2 beads were used to calibrate the system. Haemagglutination inhibition assay Antibody titres in the serum samples were determined by haemagglutination inhibition assay as described previously [9] . In brief, the serum samples were treated with receptor destroying enzyme from Vibrio cholerae by diluting one part serum with three parts enzyme and were incubated overnight in a 37 °C water bath and then were heat-inactivated at 56 °C for 30 min according to WHO’s (World Health Organization) standard procedure. Serum samples were diluted in serial twofold dilutions from 1:20 to 1:640 and then mixed with 1% suspension of chicken red blood cells and four hemagglutinating units of a local isolated virus strain A/California/07/2009 virus. Synthetic peptides A total of 893 15- to 18-mer peptides overlapping by 10 amino-acid residues and spanning the full proteome of the 2009 epidemic H1N1 influenza virus were synthesized (PEPscreen; Sigma-Aldrich) using the sequences of the A/California/04/2009(H1N1) strains. Six overlapping peptide pools representing the eight internal proteins were generated. Ex vivo interferon-γ ELISpot assay 12–16 h interferon-γ ELISpot assays were performed using cryopreserved peripheral blood mononuclear cells (PBMCs) as described previously [10] . Two lakh fifty thousand PBMCs were used in each ELISpot well in the final volume of 100 μl. The end concentration of peptide in each well was 2–3.5 μM when testing peptide pools and 2 μM when testing individual peptides. For negative and positive controls, PBMCs were incubated with media alone and with phytohemagglutinin (Wellcome), respectively. Spot forming units (SFU) were counted using an automated ELISpot reader (AID). Responses were considered positive when the number of SFU per well was greater than three times the average negative control value for the given assay, and four times the mean negative control value obtained from the peptide pool screening of all participants. Adjusted SFU after subtracting average negative values were expressed as SFUs per 1,000,000 PBMCs. Statistical analysis Statistical analysis of genetic data was performed using the χ 2 -test and the R-stats library in the R-Statistical package [11] . For association testing under different genetic models, Fisher’s exact test was additionally used since the χ 2 approximation might not hold for small samples. The Cochran-Armitage test for trend was used to test for association under the additive genetic model. Association of rs12252 to severe infection was assessed by analysing the severe infected individuals against the mildly infected individuals. The latter do not show significant differences with the Han population from 1,000 Genomes project and represent a better population-matched group for the severe infected samples. The odd ratios calculated for the association of a specific risk allele (or genotype) reflects the relative risks of the risk allele given that the incidence of severe infection is observed to be sufficiently low. PAR was estimated under the assumption that the frequency of the risk genotype (CC) in the mildly infected individuals reflected the genotype population frequency. The formula used for the PAR calculation is: PAR%=100 × p (RR−1)/ [ p (RR−1)+1], where p represents the risk genotype frequency in the population and RR represents the relative risk of the risk genotype (CC). For the calculation of the PAR for the Northern Europeans, the genotype counts of hospitalized patients and North European populations from 1,000 Genomes project were used as given in Everitt et al . [4] All other statistical analyses were performed with GraphPad Prism v 5 (GraphPad Software, San Diego, CA). Independent samples t -test were used where data were normally distributed (evaluated with Kolmogorov–Smirnov test), to compare haemagglutination inhibition levels, age, white blood cells, neutrophil counts and so on between mild and severe disease; Mann–Whitney test was used where the data were not normally distributed (MCP-1). Chi-square tests were employed to analyse the difference of gender, comorbidities, pneumonia and respiratory failure between mild and severe groups. How to cite this article: Yong-Hong Zhang et al. Interferon-induced transmembrane protein-3 genetic variant rs12252-C is associated with severe influenza in Chinese individuals. Nat. Commun. 4:1418 doi: 10.1038/ncomms2433 (2013).